Early Cretaceous chalks from the North Sea giving evidence for global change Among calcareous nannofossils, important primary producers in Jurassic and Cretaceous oceans, nannoconids were carbonate rock-forming organisms. During the late Barremian and early Aptian (~126 to 122 million years ago), nannoconids went through a crisis culminating during the Oceanic Anoxic Event 1a. Here we present nannofossil and geochemical data from a section of early Barremian–early Aptian age from the North Sea, recording the earliest chalks ever known in the Boreal Realm. These middle-late Barremian chalks were generated by blooming of endemic nannoconids under relative warm and arid conditions. A subsequent decrease of nannoconids in the latest Barremian coincides with increased nutrient and clay input. This nannoconid decline, also detected at low latitudes, was associated with the Ontong Java Plateau emplacement. We conclude that nannoconids were rock forming also at high latitudes, under clear and oligotrophic waters. Their decline was related to increased continental runoff under reinforced greenhouse conditions. Calcareous nannoplankton, and especially coccolithophores algae, are one of the most important primary producers in the marine pelagic realm and constitute the most efficient carbonate rock-forming organisms since the Jurassic. Among these, the genus Nannoconus (group incertae sedis) is represented by heavily calcified nannoliths recorded from late Jurassic and early Cretaceous sediments [1] , [2] , [3] , [4] , [5] , [6] . Nannoconids are composed of tiny calcite elements arranged around a central canal to form a cylinder or a conus. The central canal is wide or narrow and the entire structure has a size of 5–30 μm. Nannoconids have been found in the Boreal Realm and in the Tethys, Atlantic and Pacific Oceans. However, only in the Tethys they were rock-forming of Tithonian–Barremian (151–126 million years ago) [7] successions, as for example the Maiolica and Biancone Fms (Italy) [2] , [4] , [5] , [8] , [9] . Despite decades of investigations, nannoconids palaeoecology is uncertain and complete records from higher latitudes are missing. Quantitative analyses attest to a widespread decrease of nannoconids in the late Barremian (~126 million years ago) [7] , culminating with the ‘nannoconid crisis’ shortly before the deposition of the early Aptian Oceanic Anoxic Event 1a black shales [3] , [4] , [10] , [11] . This nannoconid crisis coincides with a carbonate production decline in neritic domains observed in the Tethys, Atlantic and Pacific Oceans [11] , [12] . The palaeoecological affinities of nannoconids have been discussed controversially [13] , including the following interpretations: warm waters [14] ; low nutrients [4] , [5] , [11] , [15] ; low CO 2 concentrations [4] , [6] , [10] , [11] , low terrigenous input [2] , [16] and high carbonate productivity [1] , [2] , [4] , [5] , [6] , [11] . The understanding of these affinities is crucial, as the failure of nannoconids in the late Barremian–early Aptian has been used for wide reaching, global environmental interpretations of the mid Cretaceous greenhouse world [3] , [4] , [6] , [10] , [11] , [16] . We have investigated early Barremian–early Aptian sediments of two cored wells from the North Sea, presenting a composite section ( Figs 1a , b and ). The sediments encountered comprise the earliest chalks ever known in the Boreal Realm. Calcareous nannofossil biostratigraphy and carbon-isotope data are provided and assure the age control. Quantitative data of nannofossils, temperature (TI) and nutrient (NI) indices, lithological and bulk-rock characterization are used for palaeoenvironmental and palaeoceanographic reconstructions. Our new data document that during the Barremian nannoconids were also common in the high latitudes of the Boreal Realm. Endemic taxa constitute the rock-forming organisms (abundance up to 80%) of the middle-late Barremian North Sea chalks. These nannoconid blooms are here interpreted to indicate clear waters, barren of mud, reflecting relative warm and arid conditions. The late Barremian–early Aptian nannoconid decline, now also observed in the North Sea, is ascribed to a progressive increase in nutrients and clay input, probably promoted by super-greenhouse climatic conditions imposed by volcanism of the Ontong Java Plateau. 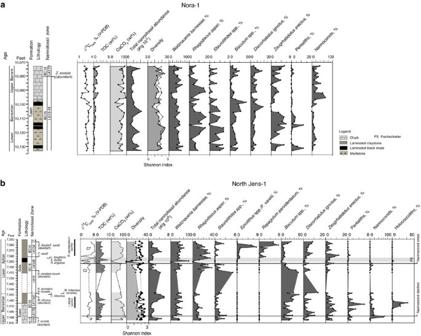Figure 1: Calcareous nannofossil and geochemistry data of the investigated wells. (a) Nora-1 core, (b) North Jens-1 core. The nannofossil zonations reported are ‘BC zones’36and ‘LK zones’16. Vertical distribution of total nannofossil abundance, and relative abundances (%) of selected taxa of calcareous nannofossils. Figure 1: Calcareous nannofossil and geochemistry data of the investigated wells. ( a ) Nora-1 core, ( b ) North Jens-1 core. The nannofossil zonations reported are ‘BC zones’ [36] and ‘LK zones’ [16] . Vertical distribution of total nannofossil abundance, and relative abundances (%) of selected taxa of calcareous nannofossils. 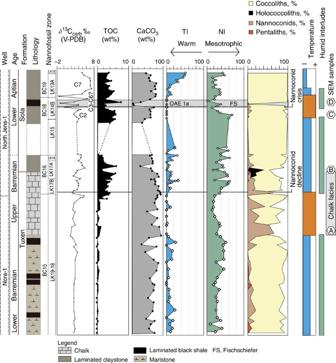Figure 2: Composite section across the early Barremian to early Aptian. The wells analysed are Nora-1 and North Jens-1. In the figure we report the carbon-isotope data, TOC (wt%), CaCO3(wt%) and calcareous nannofossil temperature (TI) and nutrient (NI) indices. The relative abundances (%) of nannoconids (in brown), coccoliths (in yellow), pentaliths (in red) and holococcoliths (in black) are also plotted. On the right, a synthesis of climatic variations is represented including temperature variations and humid interludes. Letters A to D indicate the position of the samples investigated under scanning electron microscope (Fig. 3). Full size image Figure 2: Composite section across the early Barremian to early Aptian. The wells analysed are Nora-1 and North Jens-1. In the figure we report the carbon-isotope data, TOC (wt%), CaCO 3 (wt%) and calcareous nannofossil temperature (TI) and nutrient (NI) indices. The relative abundances (%) of nannoconids (in brown), coccoliths (in yellow), pentaliths (in red) and holococcoliths (in black) are also plotted. On the right, a synthesis of climatic variations is represented including temperature variations and humid interludes. Letters A to D indicate the position of the samples investigated under scanning electron microscope ( Fig. 3 ). Full size image Biostratigraphy The biostratigraphy of both cores is based on a nannofossil scheme (LK zones) [17] , according to which the sections cover the early Barremian–early Aptian LK19 to LK12 zones ( Figs 1a , b and 2 ). Both sections overlap in correspondence of LK18 zone. Geochemistry Bulk-rock data are presented in Figs. 1 and 2 . The highest CaCO 3 content marks the upper part of the Tuxen Fm. (~80 to 100%), the lowest the Fischschiefer (5–30%). The average total organic carbon (TOC) content is 1%, highest values of 8% occur in the Fischschiefer. The δ 13 C carb values are stable for the lower part, where values of 2.7‰ are in the range of coeval sections in the North Sea [18] , Pacific [19] and Tethys [20] . Across the Fischschiefer the δ 13 C carb values decrease down to approximately −1‰. In this interval the curve is scattered indicating that for some samples diagenesis must have affected the signal. Above the Fischschiefer, the δ 13 C carb values show an increase to ~7‰ exceeding the range (4 to 5‰) detected in coeval sections [18] , [19] , [20] . In the δ 13 C carb presented segments, C2, C3–C6 and C7 of the well-established carbon-isotope curve [20] can be recognized. Calcareous nannofossils Calcareous nannofossil preservation in both cores is moderate to very good. The average Shannon Index [21] value is 1.7–2, indicating that the assemblages are moderately diversified ( Fig. 1 ). The average number of taxa detected per sample is 17. The total abundance shows no significant variations having an average of 1.11 × 10 9 (# g −1 ) for Nora-1 and 2.4 × 10 9 (# g −1 ) for North Jens-1 ( Fig. 1 ). Fluctuations in abundance of nannofossils for Nora-1, and in parentheses for North Jens-1, are described as follows: Watznaueria barnesiae has an average of 45% (36%). Biscutum constans , Zeugrhabdotus erectus and Discorhabdus ignotus are common with averages of 12% (14%), 2.4% (4%) and 6.8% (4%), respectively. Rhagodiscus asper has an average of 7% with peaks up to 16% in the uppermost part of the Tuxen Fm. and 30% just before the Fischschiefer. Holococcoliths ( Isocrystallithus dispar , Orastrum perspicuum ) are abundant (up to 40%) from 7,473.5–7,461.4 feet in North Jens-1. Peaks of pentaliths ( Micrantholithus hoschulzii, M. obtusus, M. stellatus, Braarudosphaera hockwoldensis, B. africana ) up to 5% are found in the lower part of the cored section and close to the boundary between the Tuxen and Sola Fm. Among nannoconids, the endemic species N. abundans , N. borealis , N. elongatus and N. inornatus are most abundant, followed by the cosmopolitan species N. truittii , N. circularis and N. steinmannii ( Figs 1 and 2 ). Nannoconids are abundant in LK19-18 zones where they make up around 50% (average) of the assemblages dominated by N. abundans . They decline at the base of LK17B subzone and suffer a distinctive crisis shortly before the Fischschiefer event. The absolute abundance of nannoconids is correlated with the calcium carbonate content ( R 2 =0.55). The nannofossil assemblages of the pure chalks yield abundances of up to 80%, making nannoconids the dominant nannofossil group ( Figs 2 and 3a ). The CaCO 3 content decreases by 25% between the Tuxen Fm. and the Sola Fm., accompanied by a decline of nannoconids. The highest abundances of nannoconids (0.7 × 10 9 specimens g −1 of sediment) clearly correspond to the chalk facies indicating that nannoconids were rock-forming organisms also at higher latitudes. The nannoconid decline precedes the lithological change to marls and coincides with the increase in TOC. The overlying marls show a progressive decrease in nannoconids ( Figs 2 and 3b–d ). The reminder of the calcareous nannofossils are dominated by W. barnesiae , Zeugrhabdotus spp., Biscutum spp. and D. ignotus . The presence of the latter three, dissolution prone taxa, excludes poor preservation. 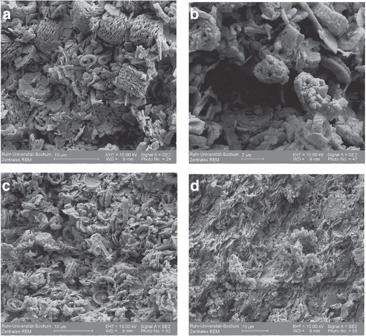Figure 3: Scanning electron microscope photos of different nannofossil assemblages. (a) Nannoconid chalk (Tuxen Fm.), (b) holococcolith-dominated assemblage (claystone, Sola Fm.), (c) coccolith-dominated assemblage (claystone, Sola Fm.), (d) coccoliths in clay matrix (Fischschiefer interval, Sola Fm.). Figure 3: Scanning electron microscope photos of different nannofossil assemblages. ( a ) Nannoconid chalk (Tuxen Fm. ), ( b ) holococcolith-dominated assemblage (claystone, Sola Fm. ), ( c ) coccolith-dominated assemblage (claystone, Sola Fm. ), ( d ) coccoliths in clay matrix (Fischschiefer interval, Sola Fm.). Full size image Fluctuations in abundance of species, selected as indicators of paleo-temperature and paleo-fertility, show patterns that justify their use in the calculation of TI and NI indices. In the Tuxen Fm., the TI indicates intermediate temperature and the NI suggests high nutrients except for the chalk interval, characterized by warmer conditions and less nutrients ( Fig. 2 ). The Sola Fm. is described by intermediate temperatures and high NI values. The Fischschiefer event is preceded by an interval of low NI coinciding with warmer temperature, the latter persisting during the Fischschiefer accompanied by high NI values. The post-Fischschiefer interval is then marked by a cooling temperature. The data set presented expands the information available for the Barremian of the North Sea area [17] , [18] , [22] , [23] . The nannoconids show fluctuations similar and coeval with those observed in the Tethys, Atlantic and Pacific [3] , [4] , [6] , [10] , including the ‘nannoconid decline’ and the ‘nannoconid crisis’ events [4] , [6] , [9] . Based on these fluctuations, and their relation to lithology and TI and NI indices, a far reaching palaeoenvironmental and palaeoceanographic reconstruction is proposed. The interval between the top of the marlstone facies of the Tuxen Fm. and the Sola Fm. is represented by chalks of the Tuxen Fm. enriched in nannoconids ( Fig. 3a ). These chalks are reflecting a reduced clastic supply, which corresponds to the onset of aridity [24] during a regressive phase. Arid conditions are associated with a lower input of continent-derived nutrients and clay minerals here in accordance with the lithology and TI and NI indices. These observations suggest that nannoconids preferred clear, clean waters, then outnumbering coccoliths. The chalks of the North Sea are coeval with Barremian limestones of the Tethys ( Fig. 4 ), which are almost entirely constituted of nannoconids (for example, Maiolica and Biancone Fms) [4] , [6] , [8] , [9] . This indicates that during a relatively brief interval across the middle-late Barremian, climatic and ecological conditions favourable for the proliferation of nannoconids were also reached in the Danish Central Trough of the North Sea. 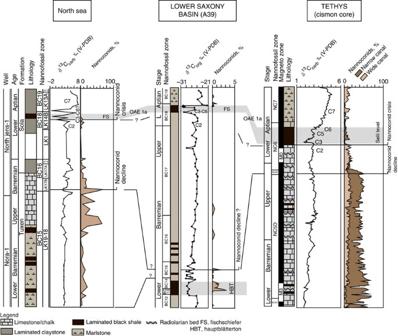Figure 4: Nannoconid abundances from various latitudes. Nannoconid relative abundances are plotted together with litho-, bio- and chemo-stratigraphy for the North Sea (Nora-1 and North Jens-1 wells, Danish Central Through, this work), Lower Saxony Basin (A39 section, Germany)27, Tethys (Cismon core, Southern Alps, Italy)6. For the Cismon, relative abundance of wide canal nannoconids are distinguished (different colours) from those of wide canal nannoconids. Figure 4: Nannoconid abundances from various latitudes. Nannoconid relative abundances are plotted together with litho-, bio- and chemo-stratigraphy for the North Sea (Nora-1 and North Jens-1 wells, Danish Central Through, this work), Lower Saxony Basin (A39 section, Germany) [27] , Tethys (Cismon core, Southern Alps, Italy) [6] . For the Cismon, relative abundance of wide canal nannoconids are distinguished (different colours) from those of wide canal nannoconids. Full size image An accelerated hydrological cycle in the late Barremian probably caused an increased input of siliciclastics and nutrients into the North Sea, thus promoting primary productivity. This environmental perturbation led to a change from pure chalk to organic-rich marl sedimentation, which went along with a shift from a nannoconid-dominated ( Fig. 3a ) to a coccolith-dominated environment ( Fig. 3c ). The transition is marked by an interval enriched in holococcoliths ( Fig. 3b ), detected also in other North Sea sites [17] , [23] . Holococcoliths are produced during the motile life stage of coccolithophore algae, but the factors inducing the secretion of holococcoliths are not well established. Stress conditions (rapid changes in surface water temperature, nutrients, light) are thought [25] to stimulate heterococcolith-bearing cells to undergo meiosis and release free motile holococcolith-bearing cells. The interval enriched in holococcoliths may thus represent further evidence of a marked change in environmental conditions. The presence of pentaliths in the same interval, considered to proliferate in coastal areas with low surface water salinity content [26] , may also reflect input of fresh water under accelerated runoff. The ‘nannoconid decline’ of the latest Barremian has been interpreted to be related to the emplacement of the Ontong Java Plateau (OJP), responsible for CO 2 emissions, input of biolimiting metals and increased nutrient supply from continental runoff under reinforced greenhouse conditions [4] , [6] , [7] , [10] , [11] , [16] . The North Sea record provides evidence for a palaeoclimatic and palaeoecological change compatible with such reconstruction, thus suggesting that the perturbation generated by OJP volcanism probably had an impact also at high latitudes. Similar lithological variations are unknown from other Boreal localities including the southernmost extension (Lower Saxony Basin) of the North Sea, where the late Barremian is represented by the Hauptblätterton (equivalent Munk Marl Bed) overlain by laminated black shales (Blätterton) and claystones. This sequence [23] , [27] is characterized by endemic nannoconids being more abundant than in the late Barremian–early Aptian [18] , [23] , [27] , [28] , but far less common than in the chalks of the Danish Central Graben. In agreement with our data, a warm climate is proposed for this time interval in the Lower Saxony Basin [28] , [29] , although accompanied by high primary productivity probably promoted by the restricted configuration of the Lower Saxony Basin. This further supports the hypothesis that nannoconid distribution was controlled by clay and nutrient input under relatively warm climate. The new calcareous nannofossil and bulk-rock data from the North Sea document that during the early and early-late Barremian common nannoconids were not restricted to the low latitudes but follow patterns similar to those detected in the Pacific, Atlantic and Tethys. Although represented by endemic forms, nannoconids were very common in the Boreal Realm, and constitute the rock-forming organisms (abundance up to 80%) of the Barremian North Sea chalks. Nannoconid blooms are here interpreted to indicate clear waters, barren of mud, reflecting relative warm and arid conditions. The ‘nannoconid decline’, now also observed in the North Sea, is ascribed to a progressive increase in nutrients and clay input recorded in the Danish Central Trough, eventually promoted by super-greenhouse climatic conditions and CO 2 emissions related to OJP volcanism. Localities The Nora-1 site is located in the centre of the Danish Central Trough. The Tuxen Formation (10,481 to 10,065 feet) is represented by marly limestones up to 10,098 feet (including the Munk Marl Bed) and by chalks up to 10,065 feet, where there is the transition to the laminated claystones of the Sola formation [30] . The North Jens-1 well was drilled 15 km southeast of the Nora-1 site. The Tuxen Fm. (7,634 to 7,466 feet) is composed of chalks and limestones, the overlying Sola Fm. (7,466 to 7,326 feet) consists of marlstones and claystones (interval 7,445 to 7,410 feet has not been recovered). The chalks of the Tuxen Fm. are homogeneous and structureless [22] , with a porosity of up to 48%. Thereby these none lithified hemi-pelagic carbonates have very good oil reservoir qualities. Consequently, several wells produce oil from the Valdemar Field in the Central Graben of the North Sea. Lithologically these Lower Cretaceous chalks resemble the Late Cretaceous (Cenomanian–Danian) chalk facies widespread in northern Europe (Denmark, northern France, Great Britain, northern Germany, North Sea, southern Sweden). A prominent laminated organic-rich unit (7,391 to 7,384 feet) corresponds to the Oceanic Anoxic Event 1a in the Boreal Realm, the Fischschiefer [22] , [31] . Sample preparation Calcareous nannofossils were investigated on settling slides of 34 samples from the Nora-1 and of 43 samples from the North Jens-1 wells. Slides were prepared following described techniques [32] . Absolute abundances of calcareous nannofossils were determined using an Olympus-BH2 light microscope with cross-polarized light at a magnification of × 1,250. At least 300 nannofossil specimens were counted in each sample. In addition, two random traverses were studied for each sample to detect rare and/or biostratigraphically important taxa. The total nannofossil abundance is expressed as number of nannofossil per gram of sediment [33] . Relative abundance of single taxa are expressed as single taxon percentage and are calculated from total nannofossil abundances. Identification of taxa is based on taxonomic guidelines [17] , [34] , [35] . The diversity of the nannoflora has been determined using the parameter of species richness and heterogeneity (Shannon Index [21] ), calculated using the software MVSP 3.1. The Shannon Index is thereby a diversity measure that takes into account both the number of species and the richness in a given data set. Calcareous nannofossils were also investigated under the scanning electron microscope for a total of six samples. Palaeoecological indices Palaeoecological indices of temperature (TI) and nutrients (NI) based on calcareous nannofossil relative abundances have been calculated for the two sections Fig. 1 . The formulas applied are modified from Tiraboschi et al . [36] who propose indices for the Aptian—Albian interval. The TI we have applied (1) excludes Z. embergeri , Rucinolithus irregularis and Manivitella pemmatoidea as they are extremely rare or not present throughout the sections. For the same reason in the formula of the NI (2) R. irregularis is excluded. Where Ss = S. stradneri; Ef=E. floralis; Rp=R. parvidentatum; Ra=R. asper; Zd=Z. diplogrammus; Bc=B. constans; Dr=D. rotatorius; Ze=Z. erectus ; Wb=W. barnesiae . Barren samples were excluded from the calculation. Geochemical analyses A total of 34 samples from Nora-1 and of 43 from North Jens-1 were investigated for TOC, CaCO 3 content and carbon isotopes. TOC analyses were performed with a Deltatronik coulometer at the Ruhr-University Bochum. The CaCO 3 content was calculated assuming the inorganic carbon measured in the samples to be in the form of CaCO 3 . Isotopic analyses on the bulk-rock were performed at the GeoZentrum Nordbayern in Erlangen (Germany) with an elemental analyzer (Carlo-Erba 1110) connected online to ThermoFinnigan Delta Plus mass spectrometer. Reproducibility of the analyses was better than ±0.06‰ (1σ). How to cite this article: Mutterlose, J. & Bottini, C. Early Cretaceous chalks from the North Sea giving evidence for global change. Nat. Commun. 4:1686 doi: 10.1038/ncomms2698 (2013).